Differentially photo-crosslinked polymers enable self-assembling microfluidics An important feature of naturally self-assembled systems such as leaves and tissues is that they are curved and have embedded fluidic channels that enable the transport of nutrients to, or removal of waste from, specific three-dimensional regions. Here we report the self-assembly of photopatterned polymers, and consequently microfluidic devices, into curved geometries. We discover that differentially photo-crosslinked SU-8 films spontaneously and reversibly curve on film de-solvation and re-solvation. Photolithographic patterning of the SU-8 films enables the self-assembly of cylinders, cubes and bidirectionally folded sheets. We integrate polydimethylsiloxane microfluidic channels with these SU-8 films to self-assemble curved microfluidic networks. Thin films with heterogeneous mechanical properties such as modulus, thickness or stress will spontaneously assemble into three-dimensional (3D) structures [1] , [2] , [3] . Several studies have sought to drive the self-assembly of polymeric thin films by inducing heterogeneities in material composition [4] , [5] , [6] . Self-assembly techniques have also previously been shown to spontaneously curve and fold two-dimensional micropatterned polymeric templates into 3D structures [7] , [8] , [9] , [10] . Yet, the self-assembly of structures with integrated microfluidic networks to enable the delivery of chemicals in curved geometries and the development of vascularized 3D systems remains a significant challenge [11] , [12] , [13] , [14] , [15] . Conventional microfluidic systems are typically built using layer-by-layer lithographic patterning methods on inherently planar substrates. Hence, although engineered microfluidic systems afford the manipulation of small liquid volumes for a variety of applications [16] , [17] , [18] , they are typically confined to block-like devices. To self-assemble microfluidic systems into 3D geometries, there is a need to develop strategies to curve and fold precisely patterned planar fluidic networks. In this work, we show how microfluidic networks can be self-assembled by integrating them with a differentially crosslinked and conditioned polymeric film. The self-assembled devices consisted of materials widely utilized in conventional microfluidics, namely polydimethylsiloxane (PDMS) and SU-8. Although stresses in SU-8 films are often undesirable [19] , [20] , [21] , we developed a strategy to create a photopatternable stress gradient in these films so that the films reversibly and reproducibly curved on solvent exchange between water and acetone. The extent and directionality of curvature was controlled by varying the ultraviolet exposure energy and direction. We could curve rectangular SU-8 structures with radii of curvature as small as 80 μm and with bidirectional curvature. We also developed a multilayer patterning scheme to integrate PDMS-based microfluidic networks with these SU-8 films and realize the self-assembly of curved microfluidic networks. Self-assembly mechanism We created heterogeneous SU-8 films with crosslink gradients (CLGs) along their thickness. SU-8 is a negative photoresist; crosslinking occurs via acid-initiated cationic polymerization on exposure to ultraviolet light and subsequent heating [21] , [22] . The extent of crosslinking within an SU-8 film can be varied by controlling the magnitude of ultraviolet exposure energy [19] , [20] , [21] . We created CLGs via low-exposure of SU-8 films to a mercury ultraviolet lamp using a commercial mask aligner without the use of optical filters that would attenuate wavelengths below 350 nm; SU-8 absorption is significant at these wavelengths ( Supplementary Fig. S1 ). This method of ultraviolet illumination resulted in progressively less exposure along the thickness of the films that caused CLGs on film baking. After exposure and baking, the photopatterned films were developed, released from the substrate, and soaked in organic solvents such as acetone to condition the films and generate a stress gradient for self-assembly. The conditioning step removed residual un-crosslinked material which we verified by comparing the dry weights of SU-8 films, before and after conditioning. We found that low-exposed SU-8 films showed a 10% decrease in weight whereas high-exposed films showed only a 1% decrease after conditioning ( Supplementary Fig. S2 ). These differentially photo-crosslinked and acetone-conditioned SU-8 films then spontaneously and reversibly curved on de-solvation by drying or the addition of water, and flattened when re-solvated by organic solvents. We attribute the spontaneous curving to a stress ( σ ) gradient formed across the thickness ( d ) of the films, arising from the CLGs and conditioning ( Fig. 1a ). SU-8 is hydrophobic and was solvated in acetone and de-solvated on drying or by the addition of water to the acetone bath. De-solvation caused a larger contraction of the lesser crosslinked portion of the film relative to the higher crosslinked portion, which caused the film to curve such that the lesser crosslinked part was concave ( Fig. 1b ). On re-solvation in acetone, the stress gradients were relieved and the film flattened ( Fig. 1c ). The process was reversible and micropatterned SU-8 films, such as an array of flower-shaped structures anchored to a glass substrate, opened and closed en masse ( Fig. 1d ). We verified reversibility of SU-8 film curving over 100 cycles and the difference (hysteresis) in the radius of curvature between the first and hundredth cycles was less than 12%. 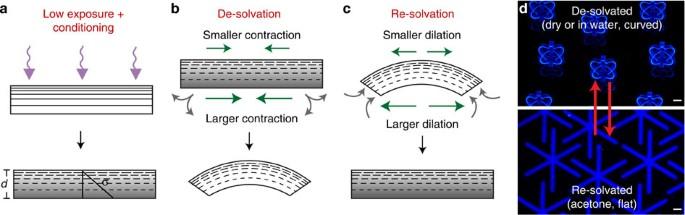Figure 1: Conceptual schematic and experimental realization of the self-assembly of differentially crosslinked and conditioned SU-8 films. (a) A schematic showing the CLG formation within a low ultraviolet exposed SU-8 film, which results in a stress (σ) gradient along the film thickness (d), on conditioning of the film in acetone to remove un-crosslinked material. (b) When water is added, the film is de-solvated and the less crosslinked side undergoes greater compression, causing the film to curve. (c) Immersion in acetone re-solvates the film, causing the film to flatten. (d) Fluorescence images of an array of flower-shaped structures that (top) reversibly curved on de-solvation and (bottom) flattened on re-solvation. Scale bars are 100 μm. Figure 1: Conceptual schematic and experimental realization of the self-assembly of differentially crosslinked and conditioned SU-8 films. ( a ) A schematic showing the CLG formation within a low ultraviolet exposed SU-8 film, which results in a stress ( σ ) gradient along the film thickness ( d ), on conditioning of the film in acetone to remove un-crosslinked material. ( b ) When water is added, the film is de-solvated and the less crosslinked side undergoes greater compression, causing the film to curve. ( c ) Immersion in acetone re-solvates the film, causing the film to flatten. ( d ) Fluorescence images of an array of flower-shaped structures that (top) reversibly curved on de-solvation and (bottom) flattened on re-solvation. Scale bars are 100 μm. Full size image We visually confirmed the formation of CLGs by fluorescence imaging of ultramicrotomed cross-sections of conditioned SU-8 films. The autofluorescence characteristic of SU-8 caused the high-crosslinked regions to fluoresce brighter than the low-crosslinked regions. Relative fluorescence intensity line plots indicated that low-exposure films exhibited a CLG, whereas high-exposure films exhibited a nearly flat relative fluorescence intensity plot ( Fig. 2a ). FTIR spectra indicated that low-exposed SU-8 films had higher fractions of epoxy groups and lower fractions of ether groups as compared with high-exposed films, confirming a lesser extent of crosslinking [21] , [23] ( Supplementary Fig. S3 ). FTIR spectra indicated not only that the chemical structure of SU-8 before and after acetone conditioning was essentially retained, but also that the photoinitiator was removed by the solvent [24] . This removal was larger for low-exposure films and increased as the acetone-conditioning time was increased ( Supplementary Fig. S4 ). 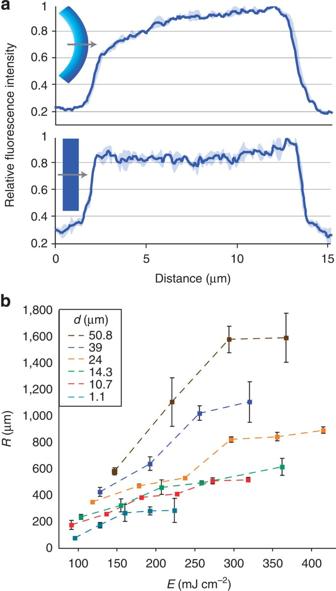Figure 2: Characterization of differentially crosslinked films. (a) Relative fluorescence intensity profiles of conditioned and sectioned SU-8 films that were ultraviolet exposed for (top) 80 mJ cm−2(32–42% of manufacturer's suggested energy) and (bottom) 300 mJ cm−2(>100% of suggested energy). Plots are averages of three lines. Shaded regions denote the standard deviation. (b) A plot of the average radius of curvature versus ultraviolet exposure energy of free-floating, self-assembled 1.5 mm×0.15 mm beams of varying film thickness.nis 6 (4 for 1.1 μm) and bars denote standard deviations. Figure 2: Characterization of differentially crosslinked films. ( a ) Relative fluorescence intensity profiles of conditioned and sectioned SU-8 films that were ultraviolet exposed for (top) 80 mJ cm −2 (32–42% of manufacturer's suggested energy) and (bottom) 300 mJ cm −2 (>100% of suggested energy). Plots are averages of three lines. Shaded regions denote the standard deviation. ( b ) A plot of the average radius of curvature versus ultraviolet exposure energy of free-floating, self-assembled 1.5 mm×0.15 mm beams of varying film thickness. n is 6 (4 for 1.1 μm) and bars denote standard deviations. Full size image Factors affecting radii of curvature We observed that the radii of curvature of conditioned SU-8 films were dependent on several controllable processing parameters: ultraviolet exposure energy, film thickness, film aspect ratio, and post-exposure bake temperature. Using a Taguchi Design of Experiments [25] , we found that ultraviolet exposure energy and film thickness most strongly affected the curvature, accounting for 76.5% of the contribution ( Supplementary Fig. S5 ). We then systematically varied the film thicknesses and exposure energies of micrometer-thick rectangular beams and measured the resulting radii of curvature after conditioning and de-solvation. The radius of curvature was found to monotonically increase as the exposure energy and film thickness were increased ( Fig. 2b ). These observations are in qualitative agreement with an optical absorption and beam mechanics model that suggests that the radius of curvature should be inversely proportional to the CLG. Details of the model can be found in Supplementary Note 1 . As described in the model, as the CLG decreases with increasing exposure energy and increasing film thickness, the radius of curvature increases accordingly. Versatility in self-assembling geometries Because the formation of CLGs was found to be ultraviolet exposure dependent, conventional photolithography afforded considerable versatility in the self-assembled 3D geometries that could be generated from initially planar templates. Through the use of multiple photomasks to differentially photo-crosslink SU-8 films from above and below, it was possible to create 3D structures with interconnected segments that either remained flat (high-exposure) or curved (low-exposure) in either direction. 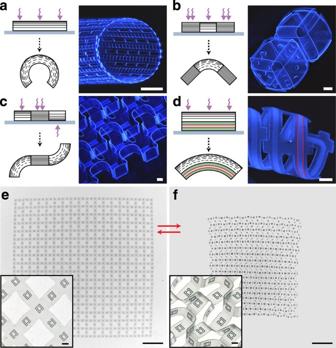Figure 3: Schematics and experimental realizations illustrating the versatility of the self-assembly methodology. (a–d) Schematics and fluorescence images of differentially photo-crosslinked and self-assembled SU-8 geometries. (a) A cylindrical mesh with hollow rectangular micropatterns and a uniform radius of curvature was self-assembled by creating a uniform CLG across the entire SU-8 film. (b) Patterned and unpatterned cubes were self-assembled with CLG hinges and flat, high-crosslinked square faces. (c) An SU-8 sheet exhibiting bidirectional curvature was self-assembled with high-crosslinked square faces and both top and bottom exposed CLG hinges. (d) A hybrid SU-8/PDMS microfluidic device was self-assembled using a CLG-containing SU-8 layer to curve an underlying PDMS channel. Red lines indicate a segment of the hollow microfluidic channel. (e,f) Brightfield images of a free-floating bidirectionally folded sheet with micrometer-scale gold SRRs patterned on the square faces. The sheet was reversibly self-assembled such that the SRRs were either (e) in a single plane when the structure flattened in acetone, or (f) arranged along thex,yandzaxes when the structure was de-solvated. Insets show magnified views of representative regions from the same film. Scale bars are 250 μm (a–d;e,finsets), 3 mm (e,f). Figure 3a–c highlights several curved or folded geometries formed in this manner: a cylindrical mesh with a uniform radius of curvature ( Fig. 3a ), cubes with flat faces and unidirectionally curved hinges ( Fig. 3b ), and a sheet with flat faces and bidirectional folds ( Fig. 3c ). Detailed process schematics of the aforementioned geometries ( Figs 1d and 3a–c ) are presented in the Supplementary Material (see Supplementary Figs S6-9 ). Figure 3: Schematics and experimental realizations illustrating the versatility of the self-assembly methodology. ( a – d ) Schematics and fluorescence images of differentially photo-crosslinked and self-assembled SU-8 geometries. ( a ) A cylindrical mesh with hollow rectangular micropatterns and a uniform radius of curvature was self-assembled by creating a uniform CLG across the entire SU-8 film. ( b ) Patterned and unpatterned cubes were self-assembled with CLG hinges and flat, high-crosslinked square faces. ( c ) An SU-8 sheet exhibiting bidirectional curvature was self-assembled with high-crosslinked square faces and both top and bottom exposed CLG hinges. ( d ) A hybrid SU-8/PDMS microfluidic device was self-assembled using a CLG-containing SU-8 layer to curve an underlying PDMS channel. Red lines indicate a segment of the hollow microfluidic channel. ( e , f ) Brightfield images of a free-floating bidirectionally folded sheet with micrometer-scale gold SRRs patterned on the square faces. The sheet was reversibly self-assembled such that the SRRs were either ( e ) in a single plane when the structure flattened in acetone, or ( f ) arranged along the x , y and z axes when the structure was de-solvated. Insets show magnified views of representative regions from the same film. Scale bars are 250 μm ( a – d ; e , f insets), 3 mm ( e , f ). Full size image Another significant advantage of this self-assembly strategy is that it is compatible with multilayer planar fabrication so that dissimilar materials, such as metals or semiconductors, can be incorporated within the differentially crosslinked SU-8 films. For example, using an extra lift-off metallization step and the same bidirectionally folded geometry shown in Figure 3c , gold split-ring resonators (SRRs) were patterned atop each of the square faces to create a reconfigurable metamaterial. A noteworthy feature of this metamaterial is that it could be reversibly folded and unfolded so that SRRs were either all periodically arrayed in the same plane (flat state; Fig. 3e ) or along each of the three ( x , y and z ) axes (folded state; Fig. 3f ). Periodic three-axis SRRs patterned within dielectric media are important optical metamaterials and are very challenging to fabricate [26] . Our self-assembly strategy also enables these materials to be reconfigured on de-solvation and re-solvation, thereby offering the possibility to create stimuli-responsive 3D metamaterials. Integration of microfluidic channels The SU-8 templates can be used as a support layer to curve thicker polymeric films and thus enables self-assembling microfluidics. 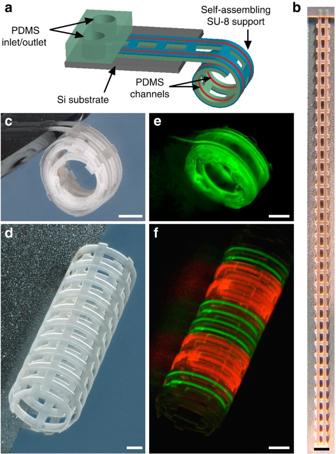Figure 4: Self-assembling microfluidic devices. (a) An illustration of a self-assembling microfluidic device with PDMS inlets/outlets attached to a Si substrate and with PDMS channels integrated with a differentially crosslinked SU-8 film. (b,c) A brightfield image of a 3.5-cm long-multilayer SU-8/PDMS microfluidic device containing a single channel, (b) as patterned on a Si substrate, and (c) after self-assembly. (d) A brightfield image of a self-assembled microfluidic device with dual channels. (e,f) Fluorescence images showing the flow of (e) fluorescein (green), and (f) fluorescein (green)/rhodamine B (red) through single and dual channel devices, respectively. Scale bars are 500 μm (1 mm forb). Shown in Figure 4a is a schematic illustration of the concept, whereby a differentially crosslinked SU-8 layer self-assembles PDMS microfluidic channels into curved 3D geometries. The overall thickness of the SU-8/PDMS devices was less than 40 μm, and they were built using planar microfabrication techniques. Multiple devices could therefore be patterned in parallel and with high resolution (for fabrication details see Supplementary Fig. S10 and Supplementary Methods ). Briefly, we sandwiched and then later dissolved sacrificial photoresist patterns between two layers of PDMS to define hollow channels. We utilized a highly crosslinked PDMS bottom layer and treated the PDMS interfaces with a low-power oxygen plasma to improve adhesion. It was also necessary to optimize the photoresist baking procedure to pattern the sacrificial resist layer without cracking. We defined inlets and outlets into the PDMS channels by using SU-8 as an etch-mask and etching away unwanted PDMS via a dry-etch plasma process [27] . Figure 4: Self-assembling microfluidic devices. ( a ) An illustration of a self-assembling microfluidic device with PDMS inlets/outlets attached to a Si substrate and with PDMS channels integrated with a differentially crosslinked SU-8 film. ( b , c ) A brightfield image of a 3.5-cm long-multilayer SU-8/PDMS microfluidic device containing a single channel, ( b ) as patterned on a Si substrate, and ( c ) after self-assembly. ( d ) A brightfield image of a self-assembled microfluidic device with dual channels. ( e , f ) Fluorescence images showing the flow of ( e ) fluorescein (green), and ( f ) fluorescein (green)/rhodamine B (red) through single and dual channel devices, respectively. Scale bars are 500 μm (1 mm for b ). Full size image To self-assemble these microfluidic devices, we released a section of the devices from the underlying silicon (Si) substrate whereas the inlets and outlets of the device remained attached to the substrate to facilitate a macro-to-micro interface. On conditioning and de-solvating the SU-8 layer, PDMS microfluidic devices as long as 3.5 cm ( Fig. 4b ) were self-assembled into cylindrical ( Figs 3d and 4c,d ) geometries. The macro-to-micro interface allowed for external control of fluid flow via syringe pumps. Flow of fluorescent liquids through the channels was visualized in both single ( Fig. 4e ) and dual ( Fig. 4f ) channel devices. We note that these hybrid SU-8/PDMS microfluidic devices reversibly self-assembled, being curved on de-solvation and flat on re-solvation. Differential photo-crosslinking of polymers advances the capabilities of self-assembly by enabling the construction and reversible reconfiguration of complex, 3D micropatterned structures. Our methodology is compatible with planar microfabrication and dissimilar materials, which is important for the self-assembly of curved optoelectronic devices [28] and the practical realization of reconfigurable 3D structural and electromagnetic metamaterials [29] . Self-assembling SU-8 films were also used to support and spontaneously curve microfluidic networks, thus enabling chemical delivery through micropatterned 3D geometries. As our methods and materials are compatible with conventional microfluidics, more complex microfluidic networks and modules could be incorporated to extend planar microfluidics to curved, thin film architectures. Another significant highlight of our methodology is that SU-8/PDMS devices are bioinert [30] , [31] , [32] , and we have verified that our self-assembled microfluidic networks remain curved in cell culture media; hence, they are relevant for biological applications. Here, we utilized fluorescent chemicals to visualize our networks as proof-of-concept, but cooling fluids and biochemical nutrients or waste could potentially be transported through these channels to create bio-mimetic self-assembled systems. Moreover, lithographically defined pores could also be incorporated along self-assembled devices to enable local release of chemicals in 3D. As many hydrogels can be photo-crosslinked [33] , [34] , [35] , [36] , [37] , it may also be possible to extend this concept towards the development of self-assembling microfluidic scaffolds for tissue engineering. Substrate preparation Soda-lime glass (Catalogue #48311-720: VWR International) and 3-inch-diameter Si wafers were used as substrates. Substrates were rinsed with deionized (DI) water, acetone and 2-propanol, and then dried with nitrogen (N 2 ) gas before use. Glass substrates allowed for bottom-side ultraviolet exposures of SU-8 films. For bottom-side exposures, a chromium (Cr) photomask was deposited onto the glass substrates via a lift-off step. Briefly, a 2.7-μm-thick layer of Microposit SC1827 photoresist (Shipley) was photopatterned, as per manufacturer's protocol, followed by thermal evaporation of a 150-nm Cr layer at a pressure of ~10 −5 torr. Dissolving the photoresist in acetone resulted in patterned Cr mask layers. Thermal evaporation of a copper (Cu) sacrificial layer atop both glass and Si substrates enabled the release of patterned films on the selective dissolution of the Cu layer in an aqueous etchant composed of 40% iron (III) chloride hexahydrate (Sigma-Aldrich) and 5% 1N hydrochloric acid [3] . A 30-nm Cu sacrificial layer (with a 5-nm Cr adhesion layer) is semi-transparent and allows for ample ultraviolet transmittance for bottom-side ultraviolet exposures through glass substrates. SU-8 photopatterning SU-8 2000 series photoresist (MicroChem) was used as received from the manufacturer. Except where specified, SU-8 2015 was spin-coated atop planar substrates at 5,000 r.p.m. for 30 s and soft-baked, as per manufacturer's protocol, yielding 10.7-μm-thick layers. Film thicknesses were measured using a DekTak IIA stylus profilometer (Veeco Instruments). All films were exposed to ultraviolet energy using a commercial mask aligner (Ultra μline Series: Quintel) fitted with a 350-Watt mercury vapour lamp (Catalogue #30273: Advanced Radiation Corporation). Because SU-8 absorbs low-ultraviolet wavelengths ( Supplementary Fig. S1 ), we exposed SU-8 films without the use of the manufacturer's recommended long-pass ultraviolet filter. Exposure energy was calculated by multiplying the ultraviolet intensity (as measured with a Vari-Wave II, 365 nm sensor: Quintel) by the exposure time. Ultraviolet intensity was measured through unpatterned substrates (photomask mounts and Cr/Cu-coated glass slides) to compensate for ultraviolet attenuation. The films were then post-exposure baked, as per manufacturer's protocol, developed for 90 s in SU-8 Developer (MicroChem) while stirring the solution at 200 r.p.m., and then rinsed with 2-propanol before drying with N 2 gas. Weight measurements Dry weight measurements of low (90 mJ cm −2 ) and high (350 mJ cm −2 ) ultraviolet-exposed SU-8 films were taken before and after the films were soaked in acetone or DI water at room temperature for 21 h ( Supplementary Fig. S2 ). The samples were dried in an oven at 100 °C for 15 min before weighing with an analytical balance (AB54-S: Mettler Toledo). Ultramicrotome SU-8 films were exposed for either low (80 mJ cm −2 ) or high (300 mJ cm −2 ) ultraviolet energy through a Cr mask to obtain micropatterned 2D sheets (similar to the mesh in Fig. 3a ). The sheets were released from the underyling substrate, rinsed with DI water, conditioned in acetone for 30 min, and desolvated on the addition of DI water. The sheets were then rinsed again with DI water before being dried, placed in empty scintillation vials, and covered with embedding resin (Catalogue #14120: Electron Microscopy Sciences) prepared by mixing the following: 200 ml Embed 812, 90 ml dodecenyl succinic anhydride, 120 ml methyl-5-norbornene-2,3-dicarboxylic anhydride, and 7 ml Ancaminek 54 curing agent. The resin-covered SU-8 sheets were desiccated overnight, pipetted into a silicone embedding mold, and then baked in an oven for ~12 h at 60 °C to harden the sectioning capsules. Sections ~250 nm in thickness were sliced using a LEICA Ultracut UCT ultramicrotome and placed on glass slides for imaging via fluorescence microscopy to visualize the crosslinking gradients ( Fig. 2a ). Fourier transform infrared spectroscopy FTIR spectra of SU-8 films were measured using a Varian 660 Spectrometer with a DTGS detector (Agilent Technologies) and dried/filtered air as the background. The spectra have a resolution of 0.4 cm −1 in the 600–4,000 cm −1 wavenumber region. The average spectrum of 256 scans was obtained using Agilent's Resolutions Pro FTIR software. Before FTIR readings, all films were released from the underlying substrate, rinsed with DI water, and dried in air. Spectra were recorded for low (90 mJ cm −2 ) and high (350 mJ cm −2 ) ultraviolet exposed films before acetone conditioning ( Supplementary Fig. S3 ). Films were also conditioned in acetone for 10 min, 3 h, or 21 h and then rinsed with DI water, dried in air, and then scanned a second time with the same settings ( Supplementary Fig. S4 ). Radius of curvature studies Taguchi Design of Experiments was implemented using the software Qualitek-4 (Nutek). An L9 array with the following four parameters and three levels were selected: ultraviolet exposure energy (150, 250, and 350 mJ cm −2 ), SU-8 thickness (1, 15, and 30 μm), photopatterned aspect ratio (1:1, 1:6, and 1:30) and post-exposure bake temperature (100, 125 and 150 °C). Curvature, which is the reciprocal of SU-8 beam radius of curvature, was used as the response parameter, and a 'larger the better' criterion was selected for the Taguchi analysis to determine which factors increased the curvature. The processing details for each of nine experiments can be found in Supplementary Table S1 . The measured data obtained over 10 trials (samples) for each of the nine experiments can be found in Supplementary Table S2 . The percent contribution of the different factors was calculated using the analysis of variance statistical method as a part of the Taguchi analysis ( Supplementary Fig. S5 ). Radius of curvature was experimentally determined for SU-8 films of varying thickness (~1–50 μm) that were photopatterned using varying ultraviolet exposure energies ( Fig. 2b ; process details can be found in Supplementary Table S3 ). The samples were ultraviolet exposed through a photomask designed with rectangular patterns of dimensions 1.5 mm×0.15 mm. After dissolving the Cu sacrificial layer, the beams were rinsed twice in DI water, rinsed once in acetone, and conditioned in acetone overnight. Curvature was induced in acetone-conditioned beams by adding DI water to the acetone (1:1 v/v). The radii of curvature were measured via bright field microscopy. Self-assembly of SU-8 geometries Detailed process schematics for each of the self-assembled SU-8 geometries presented in this work can be found in the Supplementary Material ( Supplementary Figs S6-9 ). SU-8 2015 (10.7-μm-thick) was used for each geometry. Briefly, the cylinder ( Fig. 3a ) was photopatterned using a single top-side ultraviolet exposure (120 mJ cm −2 ) through a 2D mask that defined the mesh pattern. The cubes ( Fig. 3b ) were photopatterned using two top-side exposures: a high exposure (350 mJ cm −2 ) through a mask defining the square faces, and a low exposure (90 mJ cm −2 ) through an 'overlay' mask that combined both the square faces and the curved hinges. After baking and developing the first layer of the cube template, a second layer of 10.7-μm thick SU-8 was photopatterned (350 mJ cm −2 ) atop the square faces to make them more rigid. The pattern for the bidirectional sheet ( Fig. 3c,e,f ) was adapted from prior literature [38] , [39] . Here we ultraviolet exposed a single layer of SU-8 three times: once through a photomask defining the square faces (350 mJ cm −2 ) from above, a second time through an overlay mask defining both the square faces and mountain folds (90 mJ cm −2 ) from above, and a third time through the Cr-patterned glass substrate and Cu sacrificial layer from below (90 mJ cm −2 ). Lastly, the flower array ( Fig. 1d ) was patterned using two ultraviolet exposures: a bottom-side exposure (120 mJ cm −2 ) to enable the flower petals to curve away from the glass substrate during self-assembly, and a top-side exposure (350 mJ cm −2 ) to strongly crosslink the centre of the flower. Additionally, the sacrificial layer was patterned via a lift-off step so that the flower petals could be released while the centre of each flower remained anchored to the substrate. Self-assembly of microfluidic devices For a detailed process schematic and fabrication protocol, please see Supplementary Figure S10 and the Supplementary Methods . Briefly, self-assembled microfluidic devices were fabricated by sandwiching photopatterned sacrificial photoresist channels (SC1827) between spin-coated PDMS (Sylgard 184 Silicone Elastomer Kit: Dow Corning) layers. The overall planar geometry of each self-assembled device was defined by an SU-8 layer that was photopatterned atop the PDMS; bare PDMS around the devices and atop the inlets/outlets was removed via dry-etching [27] . The SU-8 layer was patterned in registry with underlying layers. Dissolution of the Cu sacrificial layer enabled the release of the self-assembled region of the device while the base of the device (inlets/outlets) remained attached to the Si substrate to facilitate macro-to-micro interfacing. An acetone soak was used to condition the SU-8 layer and to clear the photoresist channels. Devices were self-assembled on SU-8 de-solvation, and macro-to-micro connectors were subsequently attached. How to cite this article: Jamal, M. et al . Differentially photo-crosslinked polymers enable self-assembling microfluidics. Nat. Commun. 2:527 doi: 10.1038/ncomms1531 (2011).